Phytoplankton growth after a century of dormancy illuminates past resilience to catastrophic darkness Photosynthesis evolved in the oceans more than 3 billion years ago and has persisted throughout all major extinction events in Earth's history. The most recent of such events is linked to an abrupt collapse of primary production due to darkness following the Chicxulub asteroid impact 65.5 million years ago. Coastal phytoplankton groups (particularly dinoflagellates and diatoms) appear to have been resilient to this biotic crisis, but the reason for their high survival rates is still unknown. Here we show that the growth performance of dinoflagellate cells germinated from resting stages is unaffected by up to a century of dormancy. Our results clearly indicate that phytoplankton resting stages can endure periods of darkness far exceeding those estimated for the Cretaceous-Paleogene extinction and may effectively aid the rapid resurgence of primary production in coastal areas after events of prolonged photosynthesis shut-down. Photosynthesis in the oceans is responsible for about half of the global carbon fixation. This life-sustaining process has been resilient to episodes of catastrophic environmental change across geological times. Understanding the means by which marine primary producers have survived major crises in the past might help predict their resilience to future changes. The Cretaceous-Paleogene (K-Pg) mass extinction is the most recent and well-studied biotic crisis of the Phanerozoic (last ca. 500 million years), and its evolutionary consequences extend to modern biota [1] . Strong evidence indicates that the impact of an ∼ 10-km-wide asteroid on the Earth's seafloor 65.5 million years ago ejected large amounts of material into the atmosphere, blocking sunlight to levels below photosynthesis compensation, and contributing to a global collapse of terrestrial and marine food webs [2] , [3] . The impact is expected to have resulted in massive earthquakes, widespread tsunamis, acid rain, ozone destruction and wildfires [4] , [5] , but the collapse of primary productivity is generally accepted to have been a major cause of extinction [6] . Model calculations suggest an atmospheric blackout lasting at least 6–9 months [7] , [8] , followed by a 50% drop in solar transmission for about a decade [8] . Moreover, severe cooling is expected to have altered ocean stratification and circulation for several decades, resulting in highly unstable conditions [8] . In the ocean, extinction rates between the major groups of primary producers were strikingly different, as evidenced by the fossil record [9] . Oceanic calcifying plankton (mainly coccolithophores) suffered the most drastic diversity loss ever, for example (ref. 10 ), resulting in a carbonate production crash that disrupted organic matter fluxes to the deep ocean for a period of up to 3–4 million years [11] . Much less catastrophic extinction rates were inferred from the K-Pg fossil record of coastal primary producers such as diatoms [12] and dinoflagellates [13] , [14] , [15] . In fact, life resurgence in coastal areas appears to have been relatively rapid, possibly occurring in less than a century [16] . Many modern phytoplankton species are able to combine photosynthesis with uptake of particulate food by phagocytosis, a nutritional strategy termed mixotrophy. Although mixotrophy might have been a survival advantage to some species [17] , it cannot solely explain the differential extinction. Phagotrophic mixotrophy is unknown in diatoms and some mixotrophic dinoflagellates have been reported to encyst when exposed to sudden darkness [18] . The end-Cretaceous asteroid impact is predicted to have released excessive CO 2 into the atmosphere and caused nitric- and sulphuric-acid rain [4] , [5] , [8] . Ocean acidification might have negatively affected biocalcifying organisms and has been proposed as an important cause for the near-extermination of calcareous nannoplankton, although culturing studies have shown that coccolitophores are able to maintain intracellular calcification in calcite-undersaturated waters, and can grow at low pH values [19] . A few calcareous nannoplankton survivors of the K-Pg event have recently been identified and, notably, these include species with cyst-like morphologies adapted to neritic environments [20] . Resting stages are also common among the phytoplankton groups least affected by the K-Pg extinction (diatoms and dinoflagellates). It has, therefore, been hypothesized that this life-history trait may have provided an escape from extinction [21] , [22] . In order for phytoplankton resting stages to have conferred a survival advantage at the K-Pg, these would have to remain viable for as long as the darkness and environmental instability lasted (up to several decades) and, more importantly, maintain the ability to resume vegetative growth at high rates after prolonged dormancy. Phytoplankton resting stages often result from sexual reproduction and are classically considered life-history traits to survive short-term and seasonal unfavourable conditions. They provide a seeding stock for new populations, aid dispersal, and are an import source of genetic novelty [23] . A few studies have reported survival of dinoflagellate and diatom resting stages from months to years ex situ [24] , [25] and up to several decades when naturally preserved (buried in marine sediments) [26] , [27] , [28] , but the effect of long-term dormancy on the growth performance of revived cells is unknown. Dormant stages have a highly reduced metabolism relative to actively growing vegetative cells (a 60-fold reduction was reported for the dinoflagellate Scrippsiella trochoidea ) [29] . Respiratory substrates (storage products) are used throughout the dormancy period, and resting stages also depend upon these endogenous energy reserves to germinate and become photosynthetically active [29] . Energy losses associated with long-term dormancy are, thus, expected to affect the growth performance of germinated cells. We isolated phytoplankton resting stages from sediment cores retrieved from a low-oxygen sill fjord, and found these to be viable for up to 87±12 years. We cultured strains of the dinoflagellate Pentapharsodinium dalei germinated from cysts isolated from discrete sediment core layers ( Fig. 1 ). The growth performance of the tested strains was not affected by nearly a century of dormancy. As this species belongs to a lineage well-established by the Cretaceous, and presumably little affected by the K-Pg crisis [30] , we argue that resting stages could effectively have contributed to the survival of phytoplankton groups possessing this life-history trait. Our findings indicate that resting stages in coastal sediments may play a significant role for the recovery of primary production after events of global photosynthesis disruption. 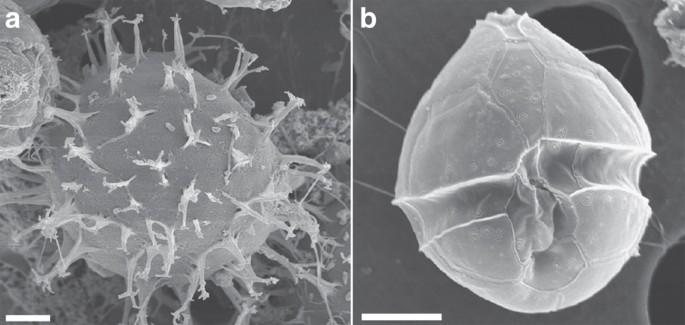Figure 1: Resting cyst and vegetative cell of the model speciesP. dalei. (a) Resting cyst isolated from coastal sediments. Scanning electron microscopy micrograph. Average resting cyst diameter=25 μm (n=15). (b) Vegetative motile stage after cyst germinations. Scanning electron microscopy. Cell length=19 μm (n=820). Scale bars in (a) and (b)=5 μm. Figure 1: Resting cyst and vegetative cell of the model species P. dalei . ( a ) Resting cyst isolated from coastal sediments. Scanning electron microscopy micrograph. Average resting cyst diameter=25 μm ( n =15). ( b ) Vegetative motile stage after cyst germinations. Scanning electron microscopy. Cell length=19 μm ( n =820). Scale bars in ( a ) and ( b )=5 μm. Full size image Sediment core chronology The age–depth model displays a linear relationship between core depth and age ( Fig. 2a ). Dry bulk density did not change markedly downcore ( Fig. 2b ), indicating relatively uniform sediment texture and compaction through time, which provides support for the reliability of the age model. The activity of unsupported 210 Pb decreased exponentially with depth ( Fig. 2c ), and was detectable down to a sediment core depth of ∼ 45 cm. The 137 Cs profile showed a distinct peak at a core depth of ∼ 10 cm that corresponds to the Chernobyl disaster of 1986 ( Fig. 2d ). The radionuclide profiles indicate that the core represents an undisturbed archive of sediments deposited through time, as supported by the laminations visible in the X-ray image ( Fig. 2e ). 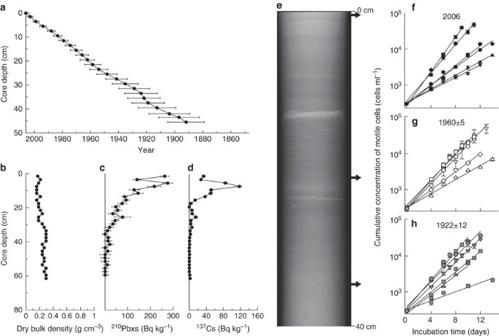Figure 2: Sediment core chronology and growth of revived cells. (a) Age–depth model for the sediment record from Koljö Fjord, resulting from a combined constant rate of supply and constant initial concentration model. Error bars are modelled standard errors. (b) Dry bulk density profile, showing relatively constant values down-core, which indicate no major changes in sediment structure or compaction through time. (c) Profile of unsupported210Pb, revealing an exponential decrease with core depth. (d) Profile of137Cs, with a distinct peak at∼10 cm, corresponding to the 1986 Chernobyl disaster. (e) X-ray radiograph of K1, revealing undisturbed laminated sediments. Arrows to the right of the X-ray image indicate the sediment layers from whichP. daleicysts were germinated for the growth experiment. (f,g) Cumulative cell concentration as a function of incubation time for the 18P. daleistrains germinated from sediment core layers dated to 2006 (f), 1,960±5 (g), and 1,922±12 (h). Errors in the dates correspond to the modelled standard errors given in (a). Different points inf–hrepresent mean values of three replicates (±standard error). Figure 2: Sediment core chronology and growth of revived cells. ( a ) Age–depth model for the sediment record from Koljö Fjord, resulting from a combined constant rate of supply and constant initial concentration model. Error bars are modelled standard errors. ( b ) Dry bulk density profile, showing relatively constant values down-core, which indicate no major changes in sediment structure or compaction through time. ( c ) Profile of unsupported 210 Pb, revealing an exponential decrease with core depth. ( d ) Profile of 137 Cs, with a distinct peak at ∼ 10 cm, corresponding to the 1986 Chernobyl disaster. ( e ) X-ray radiograph of K1, revealing undisturbed laminated sediments. Arrows to the right of the X-ray image indicate the sediment layers from which P. dalei cysts were germinated for the growth experiment. ( f , g ) Cumulative cell concentration as a function of incubation time for the 18 P. dalei strains germinated from sediment core layers dated to 2006 ( f ), 1,960±5 ( g ), and 1,922±12 ( h ). Errors in the dates correspond to the modelled standard errors given in ( a ). Different points in f – h represent mean values of three replicates (±standard error). Full size image Resting stage viability and germination We were able to revive resting cysts of P. dalei naturally preserved in the fjord sediments down to a core depth of 34 cm, corresponding to year 1,922±12 ( Fig. 2a ). Sediments deeper than 34 cm (1,922±12) were barren in viable resting cysts. Germination experiments targeted this species, but we encountered resting stages of 28 other dinoflagellate cyst taxa with visible cell contents. Viable diatoms were found in fjord sediments down to core depths corresponding to ca. 40 years of age, the non-calcifying haptophyte Isochrysis sp. was found alive after incubation of sediments dated to ca. 25 years, and filamentous cyanobacteria germinated from sediments ca. 10 years old. From a total of ∼ 450 isolated cysts, 193 Petapharsodinium dalei laboratory cultures (hereafter refereed to as strains) were established by single-cell isolation of vegetative stages germinated from individual cysts ( Fig. 1 ). All germinations took place within the first two weeks of incubation. Growth experiment Strains selected for the growth experiment were revived from three discrete sediment core layers: the surface layer, dated to 2006; an intermediate layer at 21 cm depth (1,960±5); and the layer at 34 cm depth (1,922±12) (arrows in Fig. 2e ). Germination frequency varied between 28% for the recent layer, 61% for the intermediate and 5% for the oldest layer, and more than 50 cysts were isolated from each layer. We randomly picked 18 strains for the growth experiment, comprising 6 strains revived from each of the three discrete layers. Vegetative cell concentrations increased exponentially as a function of time for all the tested strains ( Fig. 2f–h ). Balanced growth was successfully achieved, as division rates between successive samplings were nearly constant throughout the exponential growth phase. Cell division rates differed significantly among the P. dalei strains and varied between 0.17±0.07 and 0.60±0.07 day −1 (Linear Model (LM), F=4.48, d.f.=17, 225, P <2.2×10 −16 ) ( Table 1 , Fig. 2f–h ). The strain with the highest cell division rate originated from the recent layer, and the slowest from the oldest layer ( Table 1 ). Production rates, calculated as the product of division rate and cell size, also varied significantly between the strains (LM, F=264.5, d.f.=17, 11,325, P <2.2×10 −16 ; Table 1 ). The lowest and highest production rates (521±31 and 2,279±36 μm 3 day −1 , respectively) corresponded to strains germinated from the recent layer ( Table 1 ). Strain represented an important source of variation for the growth variables studied. When taking into account the random variation due to strain, no significant differences were found in cell division rates, cell size, and production rates between the three age depths tested (Linear Mixed Effects Model (LMEM), cell division rate χ 2 =0.45, d.f.=2, P =0.80; cell size χ 2 =5.63, d.f.=2, P =0.06; production rate χ 2 =1.94, d.f.=2, P =0.37; Fig. 3 ). Hence, growth performance was independent of cyst dormancy period. Table 1 Summary statistics of growth performance for the Pentapharsodinium dalei strains tested. 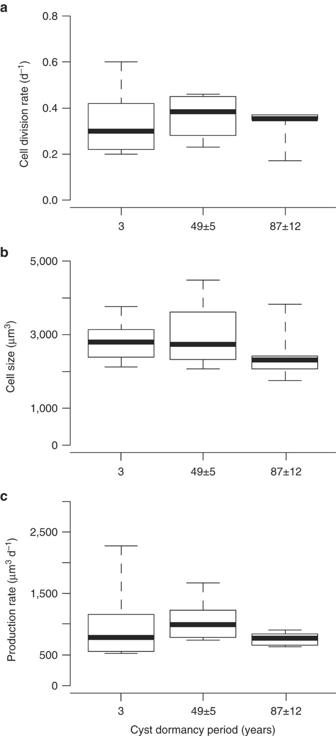Figure 3: Growth performance according to cyst dormancy period. (a) Box plots of vegetative cell division rates (day−1). (b) Cell sizes (μm3) calculated assuming the shape of an elliptical sphere, based on length and width measurements of 60 exponentially growing cells per strain. (c) Production rates (μm3day−1) calculated as the product of division rate and cell size. Lines in bold represent the median, edges of the boxes are quartiles, and whiskers indicate the maximum and minimum values. The height of the boxes indicates interquartile range and provides a measure of variability among the strains. According to maximum likelihood ratio tests of the linear mixed effects model, the mean levels were similar for the three cyst dormancy periods tested. Full size table Figure 3: Growth performance according to cyst dormancy period. ( a ) Box plots of vegetative cell division rates (day −1 ). ( b ) Cell sizes (μm 3 ) calculated assuming the shape of an elliptical sphere, based on length and width measurements of 60 exponentially growing cells per strain. ( c ) Production rates (μm 3 day −1 ) calculated as the product of division rate and cell size. Lines in bold represent the median, edges of the boxes are quartiles, and whiskers indicate the maximum and minimum values. The height of the boxes indicates interquartile range and provides a measure of variability among the strains. According to maximum likelihood ratio tests of the linear mixed effects model, the mean levels were similar for the three cyst dormancy periods tested. Full size image The quartile variation coefficient (QVC), a measure of variability, varied between the three layers (see height of the boxes in Fig. 3a–c ). The recent layer was the most diverse in terms of cell division rates (QVC=31%), and the deepest layer was the least diverse (QVC=3%), while the intermediate layer had a coefficient of 23% ( Fig. 3a ). The quartile variation coefficient of production rate was 35% for the recent layer, 22% for the intermediate and 12% for the oldest layer ( Fig. 3c ). This indicates an important drop in P. dalei growth performance variability after 49±5 years of dormancy. By germinating resting stages of the cyst-forming dinoflagellate P. dalei deposited in fjord sediments, we were able to show that the dormancy period had no reducing effect on the growth performance of revived cells. The sediment record used here was retrieved from a sill fjord experiencing recurrent anoxic conditions and virtually no bioturbation [31] . A lack of sediment disturbance was evident from the X-ray image, showing discrete laminations, and was also supported by the activity of 210 Pb and 137 Cs, providing a robust age control. In addition, any vertical contamination by smearing between layers was avoided by discarding the outer portion of each sediment layer while slicing the cores. We can therefore assume that the cysts isolated from the sediments represent, indeed, resting stages deposited in bottom sediments of the fjord over a time span from 2006 (the year of core collection) to 1,922±12. As P. dalei cysts were germinated in early 2009, we have tested growth performance after up to 87±12 years of cyst dormancy. The variation in growth parameters of P. dalei was comparable between the recent group and the group of strains revived from sediments dated to 1,960±5, but notably lower for the oldest layer (1,922±12). This drop in variability after ca. 50 years of dormancy suggests a link between the ability to optimally utilize respiratory substrates, and the ability to resume vegetative growth at high rates. This is reflected by the low germination success of the oldest layer (5%). Although a higher percentage of cysts with cell contents were no longer viable in the deepest sediment layer, those able to germinate had the same potential to actively grow in the water-column as cells germinated from recently formed cysts. For P. dalei cysts to have remained viable for nearly a century, an extremely low respiration rate and/or extensive reserves would have been needed. Carbohydrate reserves are more suitable as storage than lipids in anoxic conditions, but previous studies with dinoflagellate cysts have shown that this storage product would quickly be depleted at a constant rate of degradation [29] . Therefore, either respiration rates decrease with cyst age or other respiratory substrates (lipids or proteins) are recruited after depletion of carbohydrates [29] . The cysts retrieved from Koljö Fjord were naturally preserved in a confined environment experiencing recurrent bottom anoxia [31] . Anaerobiosis has been shown to be a crucial factor for resting cyst preservation, as it inhibits early germination without affecting cyst survival [32] . At the time of the asteroid impact, eustatic sea level was 100–200 m higher than today [33] and shallow marine environments experiencing oxygen deficiency were the rule [34] . It is, therefore, reasonable to assume that at the end-Cretaceous low-oxygen shallow environments would have provided suitable conditions for resting stage survival. The cysts isolated from Koljö Fjord sediments were able to germinate quickly after being placed at 15 °C in light and nutrient-replete conditions, regardless of dormancy period. Many studies have shown resting-stage germination to be triggered by an increase in temperature, oxygen and light conditions [23] . In the natural environment, resting stages, buried deep in the sediment, experience anoxia, darkness and lower temperatures and are unlikely to germinate unless they are brought back to the surface. This might be achieved by the movement of benthic fauna (bioturbation) or by physical processes. Impact-driven tsunamis and earthquakes are imprinted in K-Pg sediment sequences worldwide and would have had sufficient magnitude to re-suspend resting stages buried deep in shelf sediments across the globe [5] . These immediate physical processes could have transported resting stages closer to the surface, which would then contribute to the 'seed pool' after light was restored. Normal wave and current-induced resuspension of fine-grained deposits in sub- and inter-tidal environments would then provide sufficient changes in the micro-scale environment to trigger resting-stage germination [35] . Modelling studies indicate that cooling of the surface ocean would result in strong upwelling for over a decade, also leading to sediment re-suspension [8] . While screening the Koljö fjord sediments for Pentapharsodinum dalei cysts, we found viable resting stages of diatoms in sediments dated to ca. 40 years. This was not surprising, as several diatom species had previously been reported to germinate after decades of dormancy [27] , and Skeletonema marinoi over a period of more than 100 years [36] . Our observations on resting stages of other primary producers such as cyanobacteria, and non-calcifying haptophytes are relevant to discuss differential extinction, as these groups are generally not fossilizable. Our observations indicate that coastal cyanobacteria are also capable of forming resting stages that are viable for at least a decade. Many cyanobacteria produce akinetes, which are spore-like reproductive structures containing reserve material. The viability of akinetes is enhanced by low temperatures, darkness and anaerobic conditions [37] , and these can survive in lake sediments for up to 64 years [38] . A high-resolution geochemical and biomarker record from the Fiskeler K-Pg boundary layer clearly shows that whereas there was a marked decrease in chlorophyll-c-containing eukaryotic phytoplankton, cyanobacteria crossed the boundary unscathed [16] . We observed that non-calcifying haptophytes can produce resting stages able to survive in coastal sediments for at least 25 years. Isochrysis , Pavlova and Prymnesium species had previously been shown to survive in darkness, but not for periods exceeding 1 year [39] . Molecular-clock studies indicate that numerous clades of non-calcifying species with coastal affinities have survived the K-Pg extinction [40] . In contrast, calcifying (coccolitophorid) and non-calcifying oceanic clades were severely affected [10] , [40] . The fact that haptophyte resting stages have only been found in coastal species might be related to the major divergence occurring at the K-Pg between coastal and oceanic forms. Germination after long-term dormancy appears to be common for resting stages of diatoms, non-calcifying haptophytes and cyanobacteria, indicating that the ability to maintain high-growth performance, as shown here for the dinoflagellate P. dalei , is also taxonomically widespread. We, thus, propose that phytoplankton resting stages accumulated in coastal sediments have aided survival across the K-Pg and played a crucial role for the resurgence of primary production and ecosystem recovery. Phytoplankton resting stage 'banks' in coastal sediments should be incorporated in scenarios aimed at reconstructing or predicting recovery from catastrophes. It should be noted, however, that photosynthesis and biodiversity recovery do not occur at the same rates. Considering that only a fraction of modern phytoplankton groups are able to form resting stages (for example, less than 20% of modern dinoflagellate species are known to produce cysts), removing non-cyst formers at the K-Pg likely resulted in a larger diversity loss than that inferred from the fossil record (because non-cyst formers do not fossilize). Although the recovery of primary productivity after the K-Pg was relatively rapid, the recuperation in biodiversity is expected to have been delayed, due to intrinsic limits to how quickly global biodiversity can recover after extinction events [41] . The benthic realm has recently been shown to have served as an important refuge not only for primary producers but also foraminifera [42] . Benthic–pelagic coupling probably contributed to the resilience and diversification of marine life across other biological crisis in Earth history. Sediment-core sampling and dating Five sediment cores were retrieved at 45 m depth from Koljö Fjord, north of Gothenburg, Sweden (58°13′N, 11°34′E) in April 2006. This is a sill fjord with limited oxygen supply, minimum tidal activity and virtually no benthic macrofauna (resulting in nearly no bioturbation) [31] . The cores were taken with a modified micro-Kullenberg piston corer. All cores were X-rayed while intact and correlated by easily distinguishable features (lamination patterns). The cores were sliced at 1 cm intervals by extrusion from the bottom of the tube. Apart from the first sample, which had high water content, the outer 5–10 mm of each slice was scraped off to eliminate potential contamination by smearing between the layers while pushing the core upwards, and the equipment used was thoroughly rinsed between samples. The inner portion of each slice (after discarding the outer ring) was collected in individually labelled plastic bags and stored in the dark at 4 °C. Dating was based on the activity of 210 Pb, 226 Ra and 137 Cs via gamma-spectrometry measured on K4 on a Canberra low-background Germanium well detector. The activity of 210 Pb was measured via its gamma-peak at 46.5 keV, 226 Ra via the granddaughter 214 Pb (peaks at 295 and 352 keV) and 137 Cs via its peak at 661 keV. A combined constant rate of supply and constant initial concentration model [43] was applied, where the inventory below 45 cm (below the 210 Pb detection limit) was calculated on the basis of a regression. Resting stage isolation and germination To separate aggregated particles, sediment samples (ca. 5 cm 3 of wet sediment) were placed in an ultrasonic bath for 2 min, and wet-sieved with filtered seawater through a 100 μm onto a 25 μm metallic-mesh calibrated sieve. The resting stage fraction was separated from the sediments by density centrifugation (sieved aliquot added to a solution of sodium metatungstate with density 1.3 g ml −1 and centrifuged at 1,500 g for 10 min). We registered the taxonomic affinity of all resting stages encountered with cell contents (that is, potentially viable). Single resting cysts of the target species, P. dalei , were transferred with a micropipette into 96-microwell plates containing ∼ 0.25 ml of TL medium [44] . The plates were placed in a temperature controlled room at 15 °C, under an irradiance of ca. 80 μmol photons m −2 s −1 , and a light:dark cycle of 16 h:8 h. The microwells were examined for motile stages on a regular daily-to-weekly basis. Successful germinations were recorded and individual P. dalei motile cells were transferred to culture flasks and kept in TL medium under the same conditions as those for germination. A total of 193 P. dalei strains were established. Experimental conditions To test the effect of dormancy time on growth performance, we randomly picked 18 P. dalei strains revived from three discrete sediment layers (K3) dated to recent, 1,960±5 and 1,922±12. The selected strains were subjected to similar laboratory conditions until the start of the experiment. Vegetative cells were acclimated for 12 days at salinity 30 to an irradiance of 150 μmol photons m −2 s −1 , and a light:dark cycle of 16 h: 8 h. After the acclimation period, 300 vegetative cells ml −1 were transferred to fresh TL medium (pH 7.5) in closed triplicate sterile polycarbonate flasks (70 ml) filled to capacity. The 54 replicates were left to grow for 4 additional days before the first sampling for cell-concentration determination. Volumes of 5 ml were fixed with Lugol's acid and cell concentrations determined by counting at least 300 cells in Sedgewick Rafter chambers. To avoid growth limitation by increased pH due to high photosynthetic production in the closed containers [45] , we monitored pH at each sampling and assured it did not increase above the levels that affected the growth rate (<8.7). Fresh medium replaced the sample volume (5 ml). To eliminate the potential effects of slight spatial differences in irradiance, the positions of the flasks were changed randomly during the course of the experiment. Cultures used in the study are kept at the Scandinavian Culture Collection for Algae and Protozoa ( http://www.sccap.dk ). Calculations and statistics We determined cell division rates (day −1 ), cell size (μm 3 ) and production rates (μm 3 day −1 ) for the 18 tested strains. Cell division rates were calculated for each of the 54 flasks (3 replicates per strain) as the logarithm of the change in cell concentration divided by the time elapsed for each successive sampling interval (1–3 days intervals for up to 14 days of exponential growth). Cumulative cell concentrations were calculated, to account for the dilution rate (as 5 ml of sample was replaced by fresh medium at each sampling). The end of the exponential growth phase was defined as the point where the mean division rates of successively added sampling points changed in comparison to the sampling time interval day 4–8 (LM, P >0.05). Cell size was calculated assuming the shape of an elliptical sphere, based on length and width measurements of 60 exponentially growing cells per strain. Production rates were estimated as the product of cell size and division rate. To test the growth performance of revived P. dalei strains, we used a linear model of the response variables (cell division rate, cell size and production rate) as a function of strain. Accounting for random variation between the strains, we used an LMEM to study the effect of cyst dormancy period on growth performance. Initially, we modelled log-transformed cell concentrations using a 'random-slope LMEM', including all possible sources of random variation due to the variables: flask (a 54-level factor), time of sampling and strain (an 18-level factor). Random variation due to strain was ∼ 7 times higher than random variation between sampling times and no variation was explained by the random flask effect, indicating low replication error and good reproducibility in our experiment. Therefore, we chose a simplified LMEM including only the response variables (division rate, cell size and production rates) as a function of dormancy period (a 3-level factor) with strain (an 18-level factor) as a random effect. P-values were estimated based on maximum likelihood by comparing the null model including dormancy period (0-model) with the reduced nested model without the fixed effect using χ 2 -tests. The mean values (coefficients) for the three groups of strains (representing three distinct cyst dormancy periods) were calculated based on restricted maximum likelihoods. All statistical analyses were performed using R version 2.10.1 (ref. 46 ). For the LMEM we used the R package lme4 (ref. 46 ). The QVC was calculated as a means to assess the growth performance variability for each of the three cyst dormancy periods, according to the formula: QVC=100((Q3−Q1)/(Q3+Q1)), where Q1 and Q3 are the first and third quartile, respectively. How to cite this article: Ribeiro, S. et al . Phytoplankton growth after a century of dormancy illuminates past resilience to catastrophic darkness. Nat. Commun. 2:311 doi: 10.1038/ncomms1314 (2011).